Backbone-independent nucleic acid binding by splicing factor SUP-12 reveals key aspects of molecular recognition Cellular differentiation is frequently accompanied by alternative splicing, enabled by the expression of tissue-specific factors which bind to pre-mRNAs and regulate exon choice. During Caenorhabditis elegans development, muscle-specific expression of the splicing factor SUP-12, together with a member of the Fox-1 family of splicing proteins, generates a functionally distinct isoform of the fibroblast growth factor receptor EGL-15. Using a combination of NMR spectroscopy and isothermal titration calorimetry, we determined the mode of nucleic acid binding by the RNA recognition motif domain of SUP-12. The calculated structures provide the first atomic details of RNA and DNA binding by the family of proteins that include SUP-12, RBM24, RBM38/RNPC1, SEB-4 and XSeb4R. This information was further used to design strategic mutations to probe the interaction with ASD-1 and to quantitatively perturb splicing in vivo . Alternative splicing represents an important mechanism during cellular differentiation and the development of tissue, via the exclusive and timely presence of tissue-specific protein isoforms. One mechanism by which these splicing patterns are established is by the expression of splicing factors restricted to a limited stage of development or in a particular tissue. These protein factors act by enhancing or suppressing the inclusion of key exons during pre-mRNA processing. In the nematode Caenorhabditis elegans , an example of this regulated splicing involves the control of the fibroblast growth factor receptor (FGFR) gene egl-15 elicited by the muscle-specific expression of a member of the Fox-1 family in conjunction with the splicing factor SUP-12 (ref. 1 ). The egl-15 gene was initially identified as essential for sex myoblast cell migration in the developing worm [2] . Subsequent investigation revealed the presence of two alternative splice isoforms that differ in the retention of one of two mutually exclusive exons [3] , [4] . These exons (5A and 5B) are located as an atypical insertion following the N-terminal immunoglobin (IG) domain. Incorporation of exon 5B generates the essential EGL-15(5B) isoform that is required for general C. elegans development and binds to the fibroblast growth factor (FGF) LET-756. Alternative use of the downstream exon 5A produces the muscle-specific EGL-15(5A) isoform. This alternative form of the FGFR displays low affinity to LET-756 but is instead specific for EGL-17, an FGF that serves as a chemo-attractant emanating from the central gonadal cells and is required for proper migration of the sex myoblast cells from an initially anterior position. Although some details differ in mammals, this FGFR specificity switch mechanism appears to be generally conserved, as seen with the regulation of mutually exclusive exons IIIb and IIIc in the third IG domain of the homologous human FGFR2 (ref. 5 ). The binding of at least two splicing factors is required for muscle-specific isoform regulation of egl-15 . A member of the Fox-1 family of splicing factors, either FOX-1 or ASD-1, represents the first half of this regulatory switch. The Fox-1 proteins recognize conserved (U)GCAUG cis -elements within target pre-mRNA to generate isoforms specific to muscle, heart or the nervous system [6] . The main feature of this family is a central RNA recognition motif (RRM) domain characterized by a common β 1 α 1 β 2 β 3 α 2 β 4 fold, with the extended β-sheet on one side of the domain typically containing two aromatic residues involved in RNA-binding [7] . The structure of human Fox-1 (hFox-1) RRM domain bound to UGCAUGU reveals many key aspects of the molecular basis of RNA recognition for this family [8] . The second component of the splicing regulation, the protein SUP-12, also contains an RRM domain and is related to mammalian RBM24 and RBM38/RNPC1 as well as frog SEB-4 and SEB-4R [9] , [10] , [11] , [12] . In addition to egl-15 , the alternative splicing of the cofilin actin depolymerizing factor unc-60B is also regulated by SUP-12 (refs 9 , 13 ). In both cases, a sequence encompassing G-U/C-G-U-G was identified within the putative SUP-12 binding site based on conservation between the two gene targets as well as amongst several other Caenorhabditis species [1] , [13] . Furthermore, SUP-12 binding was inhibited by substitution of the middle and final guanine to cytosine [1] . However, the precise nature of the RNA sequence elements required for SUP-12 binding was not known. In addition, the details of RNA recognition, as well as potential interactions between ligand-bound SUP-12 and either ASD-1 or FOX-1, have not been investigated at the molecular level. In the current study we present structural aspects of ligand binding by the RRM domain of SUP-12, particularly in the context of egl-15 pre-mRNA alternative splicing. Atomic details are primarily derived by using NMR spectroscopy and isothermal titration calorimetry, and the molecular information is supported by in vivo measurements in live nematodes. Analysis of the structural models explains the near-equivalent binding of RNA or DNA by SUP-12 and identifies key contacts between the nucleotide bases and conserved protein residues. The presence of ASD-1 bound to an adjacent sequence motif on the egl-15 pre-mRNA results in a direct contact to the SUP-12 RRM domain but does not result in an overall increase in binding affinity. Structure of the RRM domain from SUP-12 In order to acquire molecular details of the regulation of egl-15 splicing regulation ( Fig. 1a ) we had previously characterized the secondary structure and initial RNA-binding details of the isolated RNA recognition motif (RRM) domain from SUP-12 ( Fig. 1b ; residues 28–121, hereafter SUP-12 28–121 ) [14] . To gain further insight into the molecular basis of nucleotide recognition we have determined the solution structure of the domain. The ensemble of calculated structures for the unbound sample is well defined ( Fig. 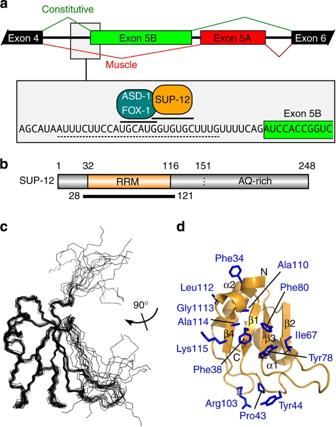Figure 1: Solution structure of the SUP-12 RRM domain. (a) Alternative splicing regulation ofegl-15. (b) Schematic diagram of full-length SUP-12 (UniProt O45189) with residue numbers indicating the boundaries of the RRM domain as well as the C-terminal location of a truncated isoform. (c) Ensemble of 15 structures calculated for the unbound SUP-1228–121. (d) Lowest energy structure of unbound SUP-1228–121in ribbon representation with labelled secondary structure elements. The location of residues predicted to be important in RNA binding based on chemical shift perturbation14are annotated and shown in blue as stick representation. The orientation compared withcis 90° as shown. Figures were made by using the PyMOL Molecular Graphics System (Schrödinger, LLC). 1c and Table 1 ) and show that SUP-12 28–121 exhibits a canonical RRM fold with a β-sheet composed of four strands opposing two α-helices on the reverse side of the domain ( Fig. 1d ). The locations of residues that experience significant chemical shift perturbation upon binding GGUGUGC RNA [14] lie in three surface regions ( Fig. 1d ), composed of residues across the β-sheet (including residues Phe38, Ile67, Tyr78 and Phe80), a region adjacent to strands β1 and β4 (Pre43, Tyr44 and Arg103), and finally N- and C-terminal residues that rest on top of the β-sheet (Phe34, Ala110, Leu112, Gly113, Ala114 and Lys115). We next wished to access further details of ligand recognition by determining the high-resolution structure of the protein-RNA complex. Unfortunately, the required high salt for protein solubility (300 mM) and unknown aspects of the complex limited the spectral quality and resulted in only a limited number of angular and distance restraints that could be obtained, thus preventing the calculation of a high-resolution structure. Figure 1: Solution structure of the SUP-12 RRM domain. ( a ) Alternative splicing regulation of egl-15 . ( b ) Schematic diagram of full-length SUP-12 (UniProt O45189) with residue numbers indicating the boundaries of the RRM domain as well as the C-terminal location of a truncated isoform. ( c ) Ensemble of 15 structures calculated for the unbound SUP-12 28–121 . ( d ) Lowest energy structure of unbound SUP-12 28–121 in ribbon representation with labelled secondary structure elements. The location of residues predicted to be important in RNA binding based on chemical shift perturbation [14] are annotated and shown in blue as stick representation. The orientation compared with c is 90° as shown. Figures were made by using the PyMOL Molecular Graphics System (Schrödinger, LLC). Full size image Table 1 NMR and refinement statistics for isolated SUP-12 28–121 and in complex with DNA or RNA. Full size table Optimization of the ligand-bound complex To obtain suitable NMR spectra we first attempted to vary buffer and temperature conditions without a noticeable improvement, and then sought to optimize the ligand itself. To provide a quantitative reference before ligand modification, we measured the affinity between SUP-12 28–121 and GGUGUGC RNA. By using isothermal titration calorimetry (ITC) under the same conditions as used for the NMR spectroscopy, we found high-affinity 1:1 binding with a K D of 69±1 nM ( Fig. 2a ). We next determined that a DNA-based scaffold with the same nucleotide sequence (GG-dU-G-dU-GC DNA) only reduced the affinity by a factor of 3.6, to give a K D value of 249±30 nM ( Fig. 2b ). This modest reduction in affinity suggests that only limited ribose-specific contacts or conformations are required to form the SUP-12 28–121 complex with RNA. Taking advantage of the high affinity of the DNA scaffold, we then tested a series of oligonucleotides based on the egl-15 sequence. By using ITC, we measured the relative affinity for 21 additional oligonucleotides in which each of the seven positions was changed to the other three bases ( Fig. 2d and Supplementary Table 1 ). The results indicate that the original sequence derived from egl-15 in fact presents a high-affinity binding motif. In addition, there is little evidence of specificity for the first and last base, suggesting that the central five bases (GUGUG) contain the critical elements of recognition. A minimal G-dU-G-dU-G DNA ligand has a reduced affinity of 843±182 nM compared with the seven-base DNA oligonucleotide, indicating that the first and/or seventh bases contribute at least partly to affinity. Unfortunately, the NMR spectra of the heptameric GG-dU-G-dU-GC or GG-dU-G-dU-G-dU DNA ligands display no significant improvement as compared with the RNA ligand. 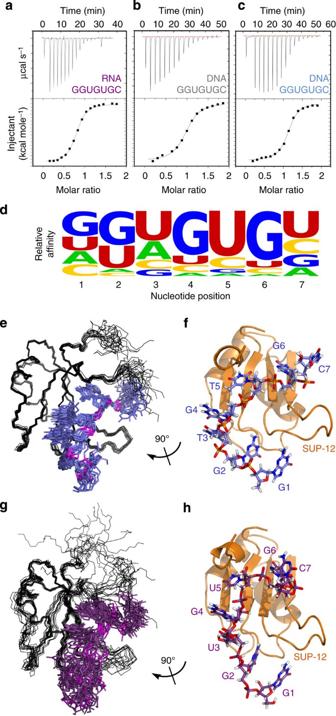Figure 2: Ligand binding by SUP-12. Affinity measurement by isothermal titration calorimetry (ITC) using (a) GGUGUGC RNA, (b) GGUGUGC DNA and (c) GGTGTGC DNA ligands. (d) Relative affinity of individual nucleotide substitutions within the GGUGUGC DNA ligand by using ITC. The height of the A (adenine), C (cytosine), G (guanine) and U (deoxyuracil) is relative to the determined values of the association constant, K (Supplementary Table 2). (e) Ensemble of 15 structures of SUP-1228–121bound to GGTGTGC DNA, along with (f) structure closest to the average. (g) Ensemble of 15 structures of SUP-1228–121bound to GGUGUGC RNA, along with (h) the structure most similar tof. Figure 2: Ligand binding by SUP-12. Affinity measurement by isothermal titration calorimetry (ITC) using ( a ) GGUGUGC RNA, ( b ) GGUGUGC DNA and ( c ) GGTGTGC DNA ligands. ( d ) Relative affinity of individual nucleotide substitutions within the GGUGUGC DNA ligand by using ITC. The height of the A (adenine), C (cytosine), G (guanine) and U (deoxyuracil) is relative to the determined values of the association constant, K ( Supplementary Table 2 ). ( e ) Ensemble of 15 structures of SUP-12 28–121 bound to GGTGTGC DNA, along with ( f ) structure closest to the average. ( g ) Ensemble of 15 structures of SUP-12 28–121 bound to GGUGUGC RNA, along with ( h ) the structure most similar to f . Full size image As a final attempt to optimize the complex, we decided to test a complete DNA ligand. Surprisingly, the affinity of GGTGTGC DNA was significantly higher than the ligand containing deoxyuracil ( Fig. 2c ). In fact, the affinity of the DNA ligand at 105±9 nM is less than twofold weaker than that of the RNA, suggesting it as a possible candidate for structure determination of the ligand-bound SUP-12 28–121 . Indeed, the quality of the NMR spectra for the GGTGTGC DNA complex displayed a significant improvement while retaining the same apparent binding mode as seen with RNA ( Supplementary Fig. 1 ). Structure of DNA-bound SUP-12 28–121 to access RNA recognition As a result of the substantial increase in spectral quality provided by the DNA ligand, we were able to measure sufficient dihedral and distance restraints for both the protein and DNA, intermolecular distance restraints and orientational restraints to calculate an ensemble of 15 high-resolution structures for SUP-12 28–121 in complex with GGTGTGC ( Table 1 and Fig. 2e ). The most notable characteristic of the DNA-bound structures is that the association is almost solely mediated by the nucleotide bases ( Fig. 2f and Supplementary Table 2 ). As described below, structural details combined with affinity measurements highlight the molecular basis of nucleic acid sequence specificity. The near-equivalent affinity for ribose or deoxyribose scaffolds suggests a shared association mechanism for the ligands, and with this in mind the DNA-bound structure was used to resolve ambiguity in the RNA-bound spectra and to guide nuclear Överhauser enhancement spectroscopy (NOESY) assignments to derive an ensemble of 15 structures for SUP-12 28–121 in complex with GGUGUGC RNA ( Table 1 and Fig. 2g ). The overall details for the RNA-bound complex are similar to that of the DNA, however, there still remains a significant reduction in precision when compared with the DNA-bound ensemble. To further confirm that the higher-resolution and more detailed structure of the bound DNA ligand provides accurate information also on the mechanism of RNA-binding, we decided to perform an investigation into the manner in which various protein mutations in SUP-12 28–121 affect the association with the three different types of ligand (RNA, deoxyuracil DNA or thymine DNA). Our choice for mutations was prompted by residues identified in a previous genetic screen (Gly40, Glu63, Ala110 and Gly113) [1] , as well as identified by chemical shift perturbation (Tyr44, Tyr78, Arg103), or located in the association surface and possessing a sidechain within a distance capable of making hydrogen bond or ionic interaction with the ligand (Lys36, His45, Lys74, Arg76, Asn97, Lys104, Asn106, Asn108). Using ITC, we observed a similar rank in affinities for the three ligands with each of the mutant proteins ( Fig. 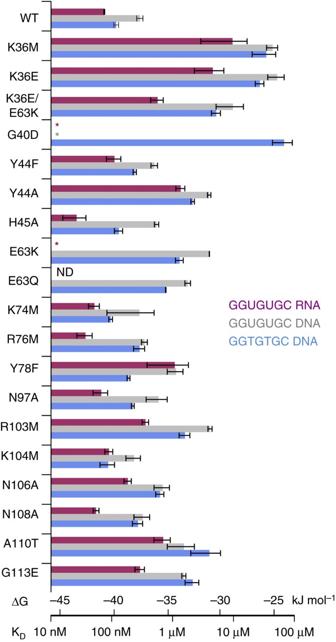Figure 3: Similarity in DNA and RNA ligand recognition. Comparison of affinities for the three ligands inFig. 2a–cfor WT SUP-1228–121as well as 19 mutant proteins. Binding is represented both in terms of free energy (ΔG) as well as KD, (seeSupplementary Table 3for values). Error from the fit to a one-site model is indicated, except for protein mutants with larger than twofold drop in affinity which show s.d. from two independent samples. In addition, error bars for the wild-type protein show s.d. based onn=4,n=7 andn=10 independent samples for the GGUGUGC RNA, GGUGUGC DNA and GGTGTGC DNA ligands, respectively. Asterisks indicate measurements that could not be fit due to weak binding (KD>10 μM). ND, not determined. 3 and Supplementary Table 3 ). For example, the mutations Y44A and R103M display a similar decrease in binding of~4 kJ mol −1 towards each of the three ligands. The only deviation from this pattern was the increased sensitivity of A110T and G113E towards the DNA ligand for reasons described below. Nevertheless, the overall evidence confirms that the DNA-bound SUP-12 28–121 recapitulates the key molecular details of the RNA-bound complex. Figure 3: Similarity in DNA and RNA ligand recognition. Comparison of affinities for the three ligands in Fig. 2a–c for WT SUP-12 28–121 as well as 19 mutant proteins. Binding is represented both in terms of free energy (ΔG) as well as K D , (see Supplementary Table 3 for values). Error from the fit to a one-site model is indicated, except for protein mutants with larger than twofold drop in affinity which show s.d. from two independent samples. In addition, error bars for the wild-type protein show s.d. based on n =4, n =7 and n =10 independent samples for the GGUGUGC RNA, GGUGUGC DNA and GGTGTGC DNA ligands, respectively. Asterisks indicate measurements that could not be fit due to weak binding (K D >10 μM). ND, not determined. Full size image Molecular details of ligand recognition Except for the last nucleotide, which is not specifically recognized by SUP-12, each base in the heptameric ligand is involved in intermolecular contacts that define the preferred sequence motif. Starting from the 5′-end of the ligand, the first two nucleotides stack upon Tyr44 ( Fig. 4b ). Interestingly, a similar mode of binding is displayed by the initial nucleotides within the complex of the hFox-1 RRM domain bound to UGCAUGU RNA [8] ( Fig. 4c ). In keeping with a role in stacking, the Y44F mutant has only a mild effect compared with wild-type ( Fig. 3 ; ΔΔG of 0.9–1.6 kJ mol −1 for the three ligands), whereas Y44A binds with significantly reduced affinity (ΔΔG of 6.1–6.8 kJ mol −1 ). Further ITC characterization of these two bases were performed by using a series of DNA ligands with both the wild-type and Y44A constructs ( Fig. 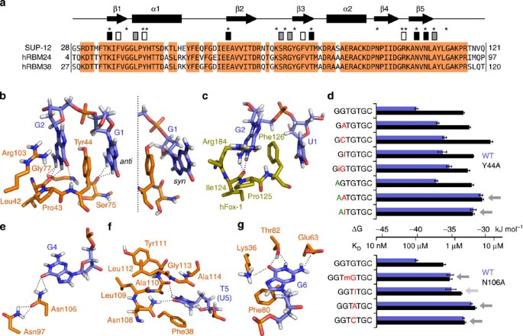Figure 4: Molecular details of nucleic acid recognition. (a) Sequence alignment showing residue identity (orange shading) betweenC. elegansSUP-12 (UniProt O45189) and the human homologues hRBM24 (UniProt Q9BX46) and hRBM38/RNPC1 (UniProt Q9H0Z9). Secondary structure based on the GGTGTGC DNA-bound SUP-1228–121is indicated above the alignment, with α-helices as cylinders and β-strands as arrows. Asterisks mark the positions of the mutated residues used in the affinity measurements (Fig. 3). Squares indicate residues involved in side-chain (black) or main-chain (grey) hydrogen bonds with the ligand, and white squares denote residues involved in stacking interactions. (b) Closeup of G1 and G2 recognition. (c) RNA recognition by human Fox-1 (PDB 2ERR). (d) ITC affinity measurements for DNA ligands with wild-type (WT), Y44A and N106 SUP-1228–121. Error from the fit to a one-site model is indicated, except for the wild-type protein with GGTGTGC DNA, which includes s.d. from 10 independent samples. Arrows point to cases in which the wild-type and mutant proteins bind the ligand with similar affinity. (e–g) Closeup of G4 (e), T5/U5 (f) and G6 (g) recognition. Molecular contacts identified by LigPlot+51and PyMOL Molecular Graphics System (Schrödinger, LLC). 4d and Supplementary Table 4 ). Replacing G2 with adenine, cytosine, inosine or iso-guanine ( Supplementary Fig. 2a ) results in a significant decrease in binding to the wild-type SUP-12 28–121 by 3.1–4.8 kJ mol −1 ( Fig. 4d , and Supplementary Table 4 ). Except for the mutation to cytosine, the G2 mutations do not cause further decreases in affinity towards the Y44A mutant. When the first base is changed to adenine, the mutation of G2 to adenine or inosine creates a ligand that has further reduced affinity, but now displays an equivalent affinity between the wild-type and Y44A mutant RRM domains. This finding confirms that Tyr44 is critical for the recognition of the first two bases, as a combination of Y44A with mutation of G1/G2 both impinge on the same binding energy. The base of G2 is also found to be in close contact with the side chain of Arg103 and a role in recognition is confirmed by ITC analysis ( Fig. 4b , Supplementary Fig. 2 and Supplementary Table 2 ). Figure 4: Molecular details of nucleic acid recognition. ( a ) Sequence alignment showing residue identity (orange shading) between C. elegans SUP-12 (UniProt O45189) and the human homologues hRBM24 (UniProt Q9BX46) and hRBM38/RNPC1 (UniProt Q9H0Z9). Secondary structure based on the GGTGTGC DNA-bound SUP-12 28–121 is indicated above the alignment, with α-helices as cylinders and β-strands as arrows. Asterisks mark the positions of the mutated residues used in the affinity measurements ( Fig. 3 ). Squares indicate residues involved in side-chain (black) or main-chain (grey) hydrogen bonds with the ligand, and white squares denote residues involved in stacking interactions. ( b ) Closeup of G1 and G2 recognition. ( c ) RNA recognition by human Fox-1 (PDB 2ERR). ( d ) ITC affinity measurements for DNA ligands with wild-type (WT), Y44A and N106 SUP-12 28–121 . Error from the fit to a one-site model is indicated, except for the wild-type protein with GGTGTGC DNA, which includes s.d. from 10 independent samples. Arrows point to cases in which the wild-type and mutant proteins bind the ligand with similar affinity. ( e – g ) Closeup of G4 ( e ), T5/U5 ( f ) and G6 ( g ) recognition. Molecular contacts identified by LigPlot+ [51] and PyMOL Molecular Graphics System (Schrödinger, LLC). Full size image Within the derived sequence motif, the uracil in position 3 has the highest tolerance for substitution ( Fig. 2d ). The presence of uracil, deoxyuracil or thymine in this position has essentially no effect on affinity ( Supplementary Table 4 ), and even the larger adenine appears to be easily accommodated without significant structural perturbation ( Supplementary Fig. 3 ). G4 in the central position is the only nucleotide in the DNA or RNA ligands that has a 3′- endo sugar conformation as confirmed by NMR spectroscopy. Nucleotides in the other positions are 2′- endo except for the final C7, which displays conformational dynamics. G4 is recognized primarily via hydrogen bonding between oxygen O6 in the base with the sidechain amide of Asn106 ( Fig. 4e ). Mutation of Asn106 to alanine results in a ΔΔG of 2.1 kJ mol −1 to the RNA or 3.9 kJ mol −1 to the DNA ligand ( Figs 3 , 4d ), consistent with the loss of a single hydrogen bond. Replacing guanine with O6-methylguanine in the GGT- m6 G-TGC DNA ligand reveals a comparable loss of 4.0 kJ mol −1 ( Fig. 4d ). Equally important, the m6 G4-containing ligand displays equivalent affinity for the both the wild-type and N106A mutant proteins ( Fig. 4d and Supplementary Table 4 ), demonstrating that the same interaction is disrupted by either the change in residue or DNA base. DNA ligands containing either C4 or A4 again have similar affinity for both the wild-type and N106A SUP-12 28–121 consistent with equivalent disruption of hydrogen bonding toward Asn106 ( Fig. 4d and Supplementary Table 4 ). An additional hydrogen bond between Asn97 and Asn106 in the ligand-bound complex further contributes to the network of interactions around G4 and explains the small decrease in affinity resulting from the mutation of Asn97 to alanine ( Fig. 3 , Supplementary Fig. 4 ). The stacking of T5 on Phe38 in strand β1 ( Fig. 4f ), and G6 onto Phe80 in strand β3 ( Fig. 4g ), both involve residues within the canonical RNP2 and RNP1 motifs, respectively, that are a common feature of RRM domains and are frequently involved in ligand binding [7] . The specificity observed for T5 or U5 is granted via hydrogen bonds, mainly by the imino H3 which is the only exchangeable hydrogen that is clearly observable for the DNA or RNA ligand and is in contact with the carbonyl from Ala110 ( Fig. 4f ). From the structural ensembles, there appears to be an additional hydrogen bond formed between oxygen O4 of T5/U5 and the sidechain amide of Asn108 ( Fig. 4f ). However, the mutant N108A does not significantly destabilize the complex ( Fig. 3 ) and therefore this second hydrogen bond may not be present at all times or is not critical to define the ligand-binding network. Unlike the canonical RRM domain, there is also a small stable C-terminal helical region in SUP-12 28–121 ( Supplementary Fig. 5 ) that packs against the β-sheet surface ( Fig. 1d ) such that it is in direct contact with the bound U5/T5 ( Fig. 2f ). Residues within the short C-terminal helix (such as Gly113 and Ala114) also contact the pyrimidine base ( Fig. 4f and Supplementary Table 2 ). The integrity of this C-terminal helix appears to be required for stability of the complex by creating an important pyrimidine-binding pocket for U5/T5, as noted by the reduced ligand binding with mutants A110T and G113E ( Fig. 3 ). 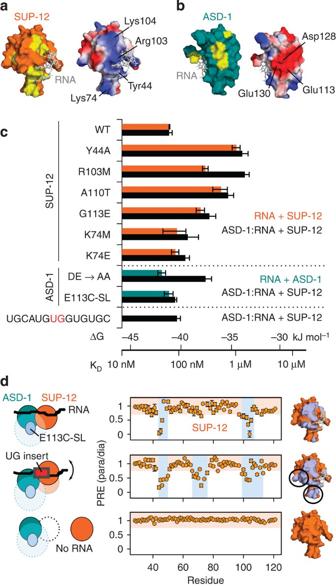Figure 5: RNA binding by SUP-1228–121in the presence of ASD-182–177. (a) Surface representation of RNA-bound SUP-1228–121highlighting the region with significant chemical shift perturbation (yellow;>1 s.d. fromSupplementary Fig. 7c) caused by the adjacent binding by ASD-182–177, with an annotated view of the putative basic patch mediating the interprotein contacts. Positive (blue) and negative (red) regions were calculated by using PyMOL Molecular Graphics System (Schrödinger, LLC). (b) Complementary interaction surface displayed on an homology model of RNA-bound ASD-182–177(>1 s.d. fromSupplementary Fig. 7b) including an annotation of the acidic patch. (c) ITC affinity measurements (Supplementary Table 6) comparing the binding of isolated SUP-1228–121and ASD-182–177to GGUGUGC (orange) or UGCAUGG (teal) RNA ligands, respectively, with affinity measurements of SUP1228–121for the longer UGCAUGGUGUGC RNA ligand (or the mutant UGCAUGUGGUGUGC) pre-bound with ASD-182–177. Error from duplicate measurements is indicated for each mutant. (d) Attachment of a paramagnetic compound to position 113 in ASD-182–177(Supplementary Fig. 8a) reveals residues in SUP-1228–121in close spatial proximity in the native complex (top), with increased separation of the RNA-binding sites (middle) and in the absence of RNA (bottom). Residues close to the spin label are observed as a reduction of NMR peak heights (paramagnetic relaxing enhancement, PRE; paramagnetic/diamagnetic <0.75) for the amide1H–15N crosspeaks, and are highlighted in blue on the surface representations of ASD-182–177and SUP-1228–121. In addition, when only T5 is changed to deoxyuracil the affinity drops to 262±44 nM ( Supplementary Table 5 ), similar to the ligand containing two deoxyuracil (249±30 nM). In contrast, replacement of T3 with deoxyuracil has little effect (144±13 nM). The stability of the DNA-bound complex is therefore particularly dependent on this hydrophobic pocket as noted by the increased sensitivity of A110T and G113E towards the GGTGTGC DNA ligand ( Fig. 3 ). G6 is recognized in the anti -conformation with hydrogen bonds observed primarily between Lys36 and atom N7, Thr82 and atom O6, as well as Glu63 and atom N2 ( Fig. 4g and Supplementary Table 2 ). This triad of residues also appear to form a stable hydrogen-bond network within the unbound SUP-12 28–121 ( Supplementary Fig. 6a ) and significant destabilization of the protein is observed when Lys36 is mutated to methionine or glutamine, with an even greater effect observed for the T82A mutation ( Supplementary Fig. 6b ). Mutations of Lys36 or Glu63 also significantly reduce affinity ( Fig. 3 ) further implicating this structured triad of residues on top of G6 in stabilizing the ligand-bound complex. RNA binding by SUP-12 adjacent to ASD-1 The binary switch from the constitutive EGL-15(5B) isoform to the muscle-specific isoform EGL-15(5A) is dependent on the presence of both SUP-12 and a member of the Fox-1 family ( Fig. 1a ). Based on previous studies [1] , a 25-nucleotide sequence was found to contain both the SUP-12 and ASD-1/FOX-1 RNA motifs ( Fig. 1a , dotted underline). The minimal hexamer UGCAUG is a well-established RNA motif for Fox-1 family proteins, and UGCAUGU was used as a high-affinity ligand in the solution structure determination of hFox-1 bound to RNA [8] . From sequence comparison, the C. elegans ASD-1 protein shares 61% identity and 76% similarity with the human homologue, including conservation of all nine residues whose sidechains directly contact RNA ( Supplementary Fig. 7a ). 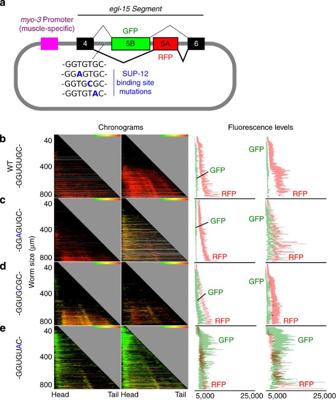Figure 6: Correlation ofin vivoalternative splicing of anegl-15-based reporter within vitromeasured affinity. (a) The mini-gene reporter based onegl-15with muscle-specific expression and exons 5B and 5A replaced with GFP and RFP, respectively15. The wild-type SUP-12 binding motif GGUGUGC is also tested as three mutated sequences based on minimal, moderate and strong binding perturbation (Supplementary Fig. 9b) Chronograms (left) and corresponding fluorescence quantification (right; arbitrary units) of exon 5B-GFP (green) and exon 5A-RFP (red) were used to determine isoform expression by using a large particle fluorescence flow cytometer (Supplementary Fig. 9a). Two independent strains are shown for each reporter, corresponding to the lowest and highest observed isoform ratios. The number of worms measured per strain are: (b, left) 9,827, (b, right) 45,172, (c, left) 19,798, (c, right) 5,691, (d, left) 52,026, (d, right) 70,105, (e, left) 9,253 and (e, right) 9,613. We produced the recombinant ASD-1 RRM domain (residues 82–177, ASD-1 82–177 ) and confirmed by using ITC high-affinity 1:1 binding to the UGCAUGG RNA sequence derived from the egl-15 pre-mRNA (52±3 nM; Supplementary Table 6 ). The adjacent and overlapping placement of the ASD-1 and SUP-12 binding sites on the egl-15 mRNA implies a direct interaction between the two RRM domains. By comparing the NMR spectra of SUP-12 28–121 bound to UGCAUGGUGUGC, without and with ASD-1 82–177 , an inter-domain surface is evident centred on an extended basic region from Arg103 and Lys104 towards Lys74 ( Fig. 5a and Supplementary Fig. 7c ). A similar analysis along with an homology model built for ASD-1 82–177 (see Methods) reveals an acidic region on ASD-1 comprising Glu113, Asp128 and Glu130 ( Fig. 5b ). Given the complementary charged surfaces on each RRM domain and the functional requirement for coordinate binding of egl-15 by ASD-1 and SUP-12, we naturally tested for cooperativity in binding. Surprisingly, we found that the affinity of SUP-12 28–121 for the 12-mer RNA pre-bound with ASD-1 82–177 was essentially equivalent to the isolated affinity of SUP-12 28–121 for the GGUGUGC RNA ligand (68±9 versus 69±1 nM, Fig. 5c and Supplementary Table 6 ). This lack of apparent cooperativity was further probed by testing several of our SUP-12 28–121 mutants. Y44A, A110T and G113E also display a similar affinity for the UGCAUGGUGUGC RNA with pre-bound ASD-1 82–177 as compared with the isolated GGUGUGC RNA ( Fig. 5c ). For the mutant R103M, there is instead an unexpected drop in affinity with the presence of ASD-1 ( Fig. 5c ). It is therefore likely that R103M creates an unfavourable interaction between the RNA-bound ASD-1 and SUP-12 that destabilizes the ternary complex. We next identified other residues that could disrupt interprotein contacts by using the identified contact regions ( Fig. 5a,b ). Mutation of Asp128 and Glu130 (DE→AA) from ASD-1 82–177 does not affect RNA-binding to UGCAUGG but indeed results in a substantial decrease towards the adjacent SUP-12 28–121 binding ( Fig. 5c ). Mutation of Lys74 on SUP-12 28–121 had only a modest decrease in affinity. Figure 5: RNA binding by SUP-12 28–121 in the presence of ASD-1 82–177 . ( a ) Surface representation of RNA-bound SUP-12 28–121 highlighting the region with significant chemical shift perturbation (yellow;>1 s.d. from Supplementary Fig. 7c ) caused by the adjacent binding by ASD-1 82–177 , with an annotated view of the putative basic patch mediating the interprotein contacts. Positive (blue) and negative (red) regions were calculated by using PyMOL Molecular Graphics System (Schrödinger, LLC). ( b ) Complementary interaction surface displayed on an homology model of RNA-bound ASD-1 82–177 (>1 s.d. from Supplementary Fig. 7b ) including an annotation of the acidic patch. ( c ) ITC affinity measurements ( Supplementary Table 6 ) comparing the binding of isolated SUP-12 28–121 and ASD-1 82–177 to GGUGUGC (orange) or UGCAUGG (teal) RNA ligands, respectively, with affinity measurements of SUP12 28–121 for the longer UGCAUGGUGUGC RNA ligand (or the mutant UGCAUG UG GUGUGC) pre-bound with ASD-1 82–177 . Error from duplicate measurements is indicated for each mutant. ( d ) Attachment of a paramagnetic compound to position 113 in ASD-1 82–177 ( Supplementary Fig. 8a ) reveals residues in SUP-12 28–121 in close spatial proximity in the native complex (top), with increased separation of the RNA-binding sites (middle) and in the absence of RNA (bottom). Residues close to the spin label are observed as a reduction of NMR peak heights (paramagnetic relaxing enhancement, PRE; paramagnetic/diamagnetic <0.75) for the amide 1 H– 15 N crosspeaks, and are highlighted in blue on the surface representations of ASD-1 82–177 and SUP-12 28–121 . Full size image With the absence of cooperative contacts between the ASD-1 and SUP-12 RRM domains, we reasoned that increased separation of their respective RNA motifs would have little detrimental effect on binding. Indeed, an addition of two intervening bases (UGCAUG UG GUGUGC) displayed comparable affinity (94±14 nM). We also wished to determine the structural consequence of this separation, especially since the guanine common to both RNA binding motifs in the native egl-15 pre-mRNA is likely bound by both proteins ( Supplementary Fig. 7d,e ). Attachment of a paramagnetic nitroxide compound to a cysteine introduced at position 113 in ASD-1 82–177 confirmed a set of residues within SUP-12 28–121 in close spatial proximity ( Fig. 5d and Supplementary Fig. 8a ). Insertion of the extra RNA bases causes increased mobility between the RRM domains as observed by a larger region affected by the nitroxide, and consistent with the absence of a single defined interaction between the two proteins. As further support for the independence of ASD-1 82–177 and SUP-12 28–121 binding, we failed to detect interaction between the isolated domains in the absence of RNA ( Fig. 5d and Supplementary Fig. 8b ). During our investigation of the 12-mer RNA, we also noted the formation of a relatively stable stem-loop (T m of 32 °C; Supplementary Fig. 8c ), that impedes binding by the first splicing protein that associates with the RNA ( Supplementary Fig. 8d,e,g ). Mutation of the ASD-1 binding motif (U CG AUGGUGUGC) also destabilizes the stem-loop and indeed allows for simple binding by SUP-12 28–121 ( Fig. 5c , Supplementary Table 6 and Supplementary Fig. 8f,g ). It is predicted that a similar stem-loop would also form with the previously characterized 25-mer ligand [1] . In vivo isoform control correlates with in vitro affinity From the in vitro data of ligand-bound SUP-12 28–121 we have an extensive description of the molecular details related to RNA binding that includes sequence requirements of the protein and RNA, as well as the apparent independent binding with respect to ASD-1 82–177 . We next aimed to determine if the association behaviour of the full-length protein in vivo correlates with the in vitro characteristics by using a fluorescent mini-gene reporter restricted to muscle expression ( Fig. 6a ) [15] . The wild-type version of the reporter recapitulates the native skipping of exon 5B in muscle cells as measured by the level of red fluorescent protein in a high-throughput assay of several thousand worms from two separate strains ( Fig. 6b ). We have used a large object flow cytometer (COPAS, Union Biometrica) to measure a high number of a varied-stage transgenic worms for green or red fluorescence representing exon 5A or 5B inclusion, respectively ( Supplementary Fig. 9a ). Using the range of binding affinities from the determination of the optimal SUP-12 sequence motif ( Fig. 2d ), we selected three additional single-base mutations with increasingly reduced affinity ( Supplementary Fig. 9b ). The strongest mutation to the sequence GGUGU A C, corresponding to a 23-fold reduction in affinity, no longer supports exon 5B skipping in keeping with the inability for SUP-12 to bind to the intron regulatory site ( Fig. 6e ). A correlated moderate effect is observed for GGUG C GC with a corresponding fourfold reduction in affinity ( Fig. 6d ). For the weakest mutation GG A GUGC (twofold drop in affinity), there is either absence or a minor effect on exon use depending on the tested strain ( Fig. 6c ). Figure 6: Correlation of in vivo alternative splicing of an egl-15 -based reporter with in vitro measured affinity. ( a ) The mini-gene reporter based on egl-15 with muscle-specific expression and exons 5B and 5A replaced with GFP and RFP, respectively [15] . The wild-type SUP-12 binding motif GGUGUGC is also tested as three mutated sequences based on minimal, moderate and strong binding perturbation ( Supplementary Fig. 9b ) Chronograms (left) and corresponding fluorescence quantification (right; arbitrary units) of exon 5B-GFP (green) and exon 5A-RFP (red) were used to determine isoform expression by using a large particle fluorescence flow cytometer ( Supplementary Fig. 9a ). Two independent strains are shown for each reporter, corresponding to the lowest and highest observed isoform ratios. The number of worms measured per strain are: ( b , left) 9,827, ( b , right) 45,172, ( c , left) 19,798, ( c , right) 5,691, ( d , left) 52,026, ( d , right) 70,105, ( e , left) 9,253 and ( e , right) 9,613. Full size image The solution structures of SUP-12 bound to RNA or DNA represent the first complete atomic descriptions of nucleic acid-bound complexes by this family of splicing factors that include human RBM24 and RBM38/RNPC1, as well as Seb4R and XSeb4 from Xenopus . Intermolecular contacts observed in the models, and further characterized by ITC, are restricted to interactions between the RRM domain and the nucleotide bases such that both ribose and deoxyribose bind with near-equivalent affinity. By using the advantageous spectral improvement due to the DNA-bound complex, we were able to calculate high-resolution models of both the DNA- and RNA-bound RRM domain of SUP-12 to identify the key aspects of nucleotide recognition. Although both SUP-12 as well as a member of the Fox-1 family are required for egl-15 alternative splicing, we did not observe any significant cooperativity towards RNA-binding affinity by their respective RRM domains. It is possible that peptide regions not included in the SUP-12 28–121 and ASD-1 82–177 constructs may mediate cooperativity in the context of the full-length proteins, or that both proteins may recognize different aspects of an auxiliary protein or complex. There may also exist a compensatory mechanism by which favourable RRM contacts counteract unfavourable aspects of ternary complex formation due to the overlapping RNA motifs, such as caused by the apparent binding of a shared guanine by both domains. Indeed, the simultaneous binding of ASD-1 and SUP-12 were negatively affected by mutations at the interface, suggesting that at least for egl-15 the complementary charged interaction regions are required to stabilize this complex. Other GU-rich binding proteins would also be unable to form these favourable contacts and therefore selectivity in the case of egl-15 may be in the inability for other splicing proteins to bind in such close proximity. Using the high-resolution structures reported in this work, comparison can be made to other RRM domains that bind to similar sequences to identify both unique aspects as well as common motifs. In the structure of CUG-BP1 RRM3 bound to UGUGUG (PDB 2RQC) [16] , the central UG is recognized by two phenylalanine in a manner similar to U5 and G6 by Phe38 and Phe80 in SUP-12 ( Fig. 4f,g ). Similar to G4 in complex with SUP-12, the preceding guanine is in the syn -conformation, however, it is the terminal amino of a lysine side chain that makes the important hydrogen bonds. The remaining bases have no counterpart in the SUP-12:RNA complex. The first two RRM domains of CUG-BP1 have also been characterized (PDB 3NNC) [17] . In the crystal structure with UUGUGUG, only the second RRM is found in complex with the RNA and once again the similarities are restricted to the central UG dinucleotide. Both nucleotides are in anti- conformation with 2′ endo sugar pucker and each are stacked onto a phenylalanine. Limited similarity to the preceding guanine lies only in a common syn -conformation with 3′ endo sugar pucker. Finally, in the complex of tandem RRM domains of TDP-43 in complex with GUGUGAAUGAAU (PDB 4BS2) [18] , the nucleotide conformation of the bound G3-U4-G5 is again similar to that of G4, G5 and G6 in complex with SUP-12, but with dissimilar types of protein contact. Interestingly, a guanine is recognized by both RRM domains reminiscent of the interface between ASD-1 and SUP-12 in the ternary complex. However, the mode of recognition by TDP-43 is not otherwise shared, and other differences include that fact that it is a single polypeptide contributing the two RRM domains and that the GU-rich motif lies instead 5′ to the shared guanine. The use of in vitro binding data in this study to predict in vivo splicing results indicate that the molecular details provide a reliable indication of biological consequence. Even the most conservative mutation to GAGUG (a twofold drop in affinity) causes altered splicing-reporter patterns in some of the corresponding strains. The strongest single base change to GUGUA still represents only a 23-fold change in K D and yet there is substantial loss in exon 5B skipping. These results suggest a relatively narrow window of tolerance for changing the affinity of the RNA sequence for SUP-12. This fact also implies that SUP-12 is unlikely to bind significantly to suboptimal RNA motifs unless cooperative interactions contribute. The narrow range in affinity would also implicate a fine control on the amount of SUP-12 protein that would be present in the target cells to regulate the muscle-specific alternative splicing. Although we did not pursue the study of protein mutations with a continuum of binding perturbation, the original characterization of the four SUP-12 mutations isolated in the genetic screen by Kuroyanagi et al. [1] , resulted in a series of worms with a variable shift from the muscle-specific form of egl-15 to the alternate isoform. Significantly, this order of phenotype effect for the four mutants (G113E<G40D, E63K, A110) correlates with a measured decrease in binding affinity to the RNA ligand GGUGUGC (K D of 246 nM for G113E, compared with 565 nM for A110T and no binding detected for G40D and E63K; Fig. 3 and Supplementary Table 3 ). A previous study to identify pentamer and hexamer sequences enriched in introns that flank alternatively spliced exons in C. elegans found a high occurrence of conserved GTGTG [19] . In particular, the sequence GTGTG was the second most frequent pentamer motif found within conserved regions adjacent to alternative exons as compared with total introns, and only the central pentamer of the Fox-1 family was more abundant. It is therefore likely that SUP-12 will contribute to alternative splicing in several genes apart from egl-15 and unc-60B . Microarray analysis using 352 alternatively spliced exons in the context of the sup-12(st89) mutant identifies mis-regulation of alternative splicing in numerous targets that indeed include an enrichment of muscle-related genes as well as a small number embryo-specific effects [20] . It is interesting to note that sup-12(st89) contains the G77E mutation which only moderately affects the in vitro binding affinity as reported above, and therefore a repeated experiment with a stronger mutant such as G40D ( yb1242 ) or E63K ( yb1278 ) may elicit the identification of additional putative targets. The atomic details described for SUP-12 also provide insight into the mode of binding by other members of this splicing factor family, with conserved residues surrounding the RNA-binding surface ( Fig. 4a ). A recent large-scale determination of RNA-binding preferences for 205 proteins suggested similar recognition motifs for SUP-12, human RBM24 and human RBM38/RNPC1 (ref. 21 ) in keeping with this surface conservation. In addition, a SELEX approach with human RBM38/RNPC1 also identified a GU-rich motif with GUGUG present in 10 of the top 15 heptamers in the final round of selection [22] . Given the increasing importance of RBM38/RNPC1 in regulating alternative splicing in human genes [22] , [23] and the role of RBM38/RNPC1 in various aspects of cancer [24] , [25] , [26] , [27] , [28] , [29] , [30] , [31] , the atomic details provided by our study of SUP-12 will provide a useful basis to understand their association mechanisms and to design strategic mutations to disrupt the function of these human homologues. In the current study we have exploited the high affinity of DNA binding to SUP-12 to counteract issues with certain NMR spectra required for structural determination. The resulting DNA-bound complex was consistent with all of the NMR spectroscopy and ITC measurements for the association with RNA, and was successfully used to generate a subsequent structure of SUP-12 bound to RNA as well as with adjacent bound ASD-1. Nevertheless, we do not rule out the possibility that the high-affinity association with single-stranded DNA could serve a specific role in C. elegans or in other species. Further experiments are required to address this speculative secondary role for SUP-12. Cloning and expression The RRM domains from C. elegans SUP-12 (residues 28–121) and ASD-1 (residues 82–177) were cloned by using PCR amplification from a cDNA library (Dualsystems Biotech). Primers were designed to introduce NcoI and Acc65I restriction enzyme sites, to allow for directional insertion into a modified pET9d vector containing an N-terminal His 6 -tag followed by a tobacco etch virus (TEV) protease cleavage site. Protein mutants were generated by using an additional set of internal PCR primers containing the mutated sequence. Plasmids were verified by sequencing and protein mutants were confirmed to be folded by using NMR spectroscopy. Protein expression in BL21(DE3)pLysY cells (Novagen) used standard media or minimal M9T media supplemented with 2 g l −1 [ 13 C]-glucose and/or 1 g l −1 [ 15 N]-ammonium chloride. Following normal growth, cells were induced at an OD 600 of ~0.6 with 0.25 μM IPTG followed by protein expression for 16 h at 25 °C. Cells were collected by centrifugation, lysed by sonication in the presence of lysozyme and then resuspended in binding buffer consisting of 50 mM Tris (pH 7.5), 500 mM NaCl, 5% (v/v) glycerol and 5 mM imidazole. The sample was added to Ni 2+ affinity chromatography resin and washed with 20 column volumes of binding buffer followed by five column volumes of the same buffer but with 30 mM imidazole. Elution with 50 mM Tris (pH 7.5), 500 mM NaCl, 5% (v/v) glycerol and 250 mM imidazole was followed by a buffer exchange to 20 mM sodium phosphate (pH 6.5) and 300 mM NaCl using a PD10 column (GE Healthcare). After cleavage with TEV protease for 16 h at 22 °C, the TEV protease, His 6 -tag and uncleaved protein were removed via a second passage of the sample through Ni 2+ affinity chromatography resin. The eluate was concentrated to at least 0.2 mM protein using a Vivaspin (Sartorius) centrifugal filter unit with 5,000 Da molecular weight cutoff. Oligonucleotides DNA oligonucleotides for cloning and as ligands were purchased from MWG Biotech (Munich, Germany). RNA oligonucleotides were purchased from Biospring GmbH (Frankfurt, Germany) and Eurogentec (Angers, France). NMR spectroscopy Samples contained between 0.2 to 2 mM protein in 20 mM sodium phosphate (6.5), 300 mM NaCl, 2 mM dithiothreitol and either 10 or 99% 2 H 2 O. NMR experiments were conducted at a temperature of 298 K on a triple resonance Bruker Avance 700 MHz, as well as a cryoprobe-equipped Bruker Avance 800 MHz. Spectra were processed using NMRPipe/Draw [32] and analysed using Sparky 3 (T. D. Goddard & D. G. Kneller, University of California, San Francisco, USA). Chemical shift assignment Backbone and aliphatic sidechain assignments for isolated SUP-12 28–121 and for SUP-12 28–121 bound to GGUGUGC RNA were already described [14] . Assignments for SUP-12 28–121 bound to GGTGTGC DNA were obtained from two-dimensional (2D) 13 C- and 15 N-HSQC, 2D and three-dimensional (3D) HNCO, 3D HNCACO, 3D HNCA, 3D HNCOCA, 3D HNCACB, 3D CBCA(CO)NH, 3D HCACO, 3D (H)CC(CO)NH-TOCSY, 3D H(CC)(CO)NH-TOCSY, 3D HC(C)H-TOCSY and 3D (H)CCH-TOCSY spectra. Aromatic resonances were assigned from 2D 13 C-HSQC, 2D 15 N-HMBC, 2D DQF-COSY, 2D 1 H, 1 H-NOESY, 2D HBHD and 2D HBHE spectra. Glutamine and asparagine sidechain amides were assigned using spectra from a 3D HNCO, 3D HNCACB, 3D CBCA(CO)NH and confirmed using a 3D 15 N-NOESY (120 ms mixing time). Stereospecific assignments for valine and leucine methyl groups were achieved using a 2D constant-time 13 C-HSQC and a 10% uniform- 13 C labelling scheme [33] . DNA assignments were based on double-filtered 2D 1 H, 1 H-TOCSY (40 and 120 ms mixing times) and 1 H, 1 H-NOESY (120 ms mixing time) spectra on a sample of 13 C, 15 N-labelled SUP-12 28–121 in complex with unlabelled ligand, as well as 2D 13 C-HMQC and 2D 15 N-HSQC spectra with site-specific incorporation of 13 C, 15 N-labelled nucleotides by using chemically synthesized DNA. Backbone 1 H, 13 C and 15 N nuclei for SUP-12 28–121 or ASD-1 82–177 bound to UGCAUGGUGUGC RNA, as well as SUP-12 28–121 and ASD-1 82–177 within the ternary complex were based on additional 3D HNCO and 3D HNCACB spectra. ASD-1 assignments were further assisted by comparison with 3D HNCO, 3D HN(CA)CO, 3D HNHA and 3D HNCACB spectra collected on the unbound ASD-1 82–177 . Structure calculation The three ensembles of structures were calculated by using a standard ARIA 1.2/CNS 1.1 setup [34] , [35] , [36] . For the unbound SUP-12 28–121 , proton distances were obtained from a 3D 1 H, 15 N-HSQC-NOESY (120 ms mixing time) and a 3D 1 H, 13 C-HSQC-NOESY (120 ms mixing time). An initial set of 2,509 manually-assigned distance restraints was accompanied by 283 peaks with ambiguous assignment. Hydrogen bond restraints (two per hydrogen bond) were included for amides that displayed reduced exchange with 2 H 2 O and were within a clearly identified secondary structure. Dihedral angles were obtained from TALOS+ (ref. 37 ), with the error twice that predicted. Leucine χ angles were only used when 13 C δ1 and 13 C δ2 values were indicative of a single rotamer [38] . The 15 lowest energy structures following the final water refinement of 100 structures were taken as the calculated ensemble. Using PROCHECK-NMR [39] , there are 90.3% of residues in the most favoured and 9.7% of residues in additional allowed regions, for the residues from Thr32 to Pro116, and there were no outliers. For the DNA-bound SUP-12 28–121 , proton distances were obtained from a 3D 1 H, 15 N-HSQC-NOESY (120 ms mixing time), 3D 1 H, 13 C-HSQC-NOESY (120 ms mixing time), a 13 C, 15 N double-filtered 2D 1 H-NOESY spectra (120ms mixing time), and a 2D 1 H-NOESY spectra (120ms mixing time) with a 13 C, 15 N filter only applied in the direct dimension. An initial set of 3,721 manually-assigned distance restraints was accompanied by 564 peaks with ambiguous assignment. Hydrogen bond restraints (two per hydrogen bond) were included for amides that displayed reduced exchange with 2 H 2 O and were within a clearly identified secondary structure. Backbone and χ 1 dihedral angles were obtained from TALOS-N [40] , with the Φ and Ψ and error twice that predicted, and χ 1 errors set to 15°. Leucine χ angles were only used when 13 C δ1 and 13 C δ2 values were indicative of a single rotamer [38] . 1 H– 15 N residual dipolar couplings were measured using an interleaved spin state-selective 1 H, 15 N-TROSY experiment, without and with a liquid crystalline mixture of hexanol and pentaethylene glycol monododecyl ether [41] . Residual dipolar couplings for residues with { 1 H} 15 N heteronuclear NOE values >0.6, were incorporated starting at iteration four, and used Da and R -values of 13.0 and 0.25, respectively. The 15 lowest energy structures following the final water refinement of 100 structures were taken as the calculated ensemble. Using PROCHECK-NMR [39] , there are 95.4% of residues in the most favoured and 4.5% of residues in additional allowed regions for the protein residues from Thr32 to Pro116, with only one outlier in the ensemble in the disallowed region. The RNA-bound SUP-12 28–121 structure calculation relied on proton distances obtained from a 3D 1 H, 13 C-HSQC-NOESY (120 ms mixing time), a 13 C, 15 N double-filtered 2D 1 H-NOESY spectra (300 ms mixing time), and a 2D 1 H-NOESY spectra (300 ms mixing time) with a 13 C, 15 N filter only applied in the direct dimension. An initial set of 2,373 manually-assigned distance restraints were included, using comparison to the spectra from the DNA-bound complex to resolve a significant amount of assignment ambiguity especially for the RNA intra- and intermolecular restraints. Five hundred and fourteen peaks with ambiguous assignment were also included. Hydrogen bond restraints for backbone amides (two per hydrogen bond) were based on the DNA-bound structure. Backbone and χ 1 dihedral angles were obtained from TALOS-N [40] , with the Φ and Ψ and error twice that predicted, and χ 1 errors set to 15°. 1 H– 15 N residual dipolar couplings were measured for the same range of residues as defined for the DNA-bound complex, and were incorporated starting at iteration four using Da and R -values of 13.0 and 0.25, respectively. Sugar conformation was confirmed by the observation of a strong TOCSY crosspeak between H1′ and H2′ for all nucleotides except G4, with determination of syn / anti -based on the double-filtered NOESY spectrum. The 15 lowest energy structures following the final water refinement of 125 structures were taken as the calculated ensemble. There are 85.2% of residues in the most favoured and 13.2% of residues in additional allowed regions by using PROCHECK-NMR [39] for the protein residues from Thr32 to Pro116, with 0.9 and 0.7% of residues in the generously allowed and disallowed regions, respectively. Homology model of the RRM domain from ASD-1 The method used to calculate the model ASD-1 82–177 was based on a semi-rigid body assembly protocol as previously described [42] , [43] . For ASD-1 82–177 , a homology model was first created based on the structure of hFox-1 bound to RNA (PDB 2ERR) [8] by using SWISS-MODEL [44] , [45] , [46] . The overall fold of ASD-1 82–177 was maintained by using a weighting factor of 10 for the non-crystallographic symmetry term within CNS/ARIA for residues 99 to 172 of the homology model structure. The structure was further optimized during refinement by the addition of 41 hydrogen bonds (via 82 distance restraints) obtained by analogy to the Fox-1 structure, as well as 71 Φ, 71 Ψ and 34 χ 1 dihedral angle restraints derived from TALOS-N [40] analysis of the chemical shift assignments of RNA-bound ASD-1 82–177 . The UGCAUGG RNA ligand was left random regarding the non-crystallographic symmetry term. For the RNA bases U1 to G6, the chemical shift values and NOESY patterns were similar to those of the RNA bound to hFox-1, consistent with a mode of RNA binding conserved between the two proteins. A set of 86 intra- and 220 intermolecular restraints towards ASD-1 were derived based on heavy-atom distances observed for the RNA-bound Fox-1 structure, to preserve the general conformation of the RNA ligand as well as the details of protein-RNA recognition. The hydrogen bonds between G2 and A4 were also included. Paramagnetic relaxation enhancement Three residues on the surface of ASD-1 82–177 (Glu113, Asn148 and Asn160) and three on SUP-12 28–121 (His45, Asn71 and Asp95) were independently mutated to cysteine. After protein expression, purification and addition of 4 mM dithiothreitol, the buffer was changed to 20 mM Tris (pH 8.0) with 150 mM NaCl. Five molar equivalents of 4-(2-iodoacetamido)-2,2,6,6,tetramethyl-1-piperidinyloxy (TEMPO) free radical dissolved in methanol were added to the samples followed by an overnight incubation in the dark at 4 °C. The modified proteins were concentrated and then extensively dialyzed in 20 mM sodium phosphate (pH 6.5) and 300 mM NaCl. Of the six samples, SUP-12 28–121 (H45C) was not accessible to modification. ASD-1 82–177 (E113C)-TEMPO resulted in significant paramagnetic relaxation enhancement towards both proteins, whereas the remaining four had only limited interprotein effects. 15 N relaxation measurement Amide 15 N relaxation data were acquired at 700 MHz and 298 K as described [47] . Steady-state heteronuclear { 1 H} 15 N-NOE spectra were recorded with and without 3 s of 1 H saturation. Relaxation rates and error calculations were determined using NMRViewJ [48] . Isothermal titration calorimetry Isothermal titrations were conducted at 25 °C using an ITC200 Microcalorimeter from Microcal, (Northhampton, USA). All proteins were dialyzed extensively against 20 mM sodium phosphate (pH 6.5) and 300 mM NaCl. Buffer from the dialysis was used to resolubilize the RNA and DNA oligonucleotides and to provide a baseline as required. The data were analysed using Origin version 5.0 provided by Microcal using a one-site model. The concentrations used in the ITC cell are in the range of 2 to 5 μM for the RNA sequences and 5 to 10 μM for the DNA sequences. The concentrations of ASD-1 and SUP-12 proteins inside the syringe were between 30 and 100 μM. Following an initial injection of 1.5 μl, a total of 15 injections of 2 μl were performed. The initial delay was set to 120 s, and the delay between each titration point was 180 s. Sensitivity was set to normal and a value of 6, and the reaction mixture was constantly stirred at 600 r.p.m. Thermal denaturation Ultraviolet-melting measurements were performed on a Cary100 ultraviolet/visible spectrophotometer (Agilent Technologies) equipped with a Pelletier temperature-control accessory. The oligonucleotide was solubilized in 20 mM sodium phosphate (pH 6.5) and 300 mM NaCl at a final concentration of 5 μM. A temperature-increase rate of 0.2 °C min −1 was applied and the absorbance values were measured every 1 °C. The temperature was determined with an inert glass sensor immersed into a quartz cell filled with water. The absorbance was monitored at 260, 273 and 280 nm using a quartz cell of 1 cm path length and 600 μl of volume. Nematode transgenesis Wild-type C. elegans obtained from the Caenorhabditis Genetics Centre (NIH) at stage N2 were microinjected with 50 ng of reporter construct plasmid (encoding GUGUG, GAGUG, GUGCG or GUGUGA in the SUP-12 binding site) and 10 ng of plasmid pRG02 (carrying the neomycin resistance gene). The reporter plasmid pmyo3-EGL-15-BGAR [1] was provided by H. Kuroyanagi (Tokyo Medical and Dental University) and subsequently mutated by using the QuikChange protocol (Stratagene) and verified by DNA sequencing. Injected P0 were placed on NGM plates with 0.4 mg ml −1 G418 and left to proliferate to select for successfully transformed progeny [49] . After 3 to 6 days F1 adults were isolated on fresh selective plates. For each construct, two to three independent lines carrying the antibiotic resistance were isolated from these independent progenitors. In vivo fluorescence measurement Mixed-stage populations of at least 5,000 transgenic nematodes were measured by using the COPAS-Profiler2 (Union Biometrica). Absolute value of fluorescence for individual worms are represented, and worms were only included if at least one fluorescence channel was above background. Individual worm profiles were then assembled into chronograms to visualize the ratio of fluorescence of each of the reporters along the animal body during the postembryonic development as previously described [50] . Each line of a chronogram represents the average profile of all the worms of the same exact size in the population analysed (see Supplementary Fig. 9a for schematic). As the animals pass through the profiler either tail or head first, all profiles are oriented relative to one another by using an automated method based on the best fit with their neighbours as determined by Pearson’s correlation coefficient [50] . Accession codes: Coordinates for the structures have been deposited in the Protein Data Bank under accession codes 4CH0 , 4CH1 and 4CIO for the unbound, DNA-bound and RNA-bound SUP-12 28–121 , respectively. The chemical shift assignments for the DNA-bound SUP-12 28–121 , unbound ASD-1 82–177 and RNA-bound ASD-1 82–177 have been deposited in the Biomolecular Magnetic Resonance Data Bank under accession codes 19653 , 19680 and 19686 , respectively. How to cite this article: Amrane, S. et al. Backbone-independent nucleic acid binding by splicing factor SUP-12 reveals key aspects of molecular recognition. Nat. Commun. 5:4595 doi: 10.1038/ncomms5595 (2014).